NCR+ILC3 concentrate in human lung cancer and associate with intratumoral lymphoid structures Tertiary lymphoid structures (TLSs) are a common finding in non-small cell lung cancer (NSCLC) and are predictors of favourable clinical outcome. Here we show that NCR + innate lymphoid cell (ILC)-3 are present in the lymphoid infiltrate of human NSCLC and are mainly localized at the edge of tumour-associated TLSs. This intra-tumoral lymphocyte subset is endowed with lymphoid tissue-inducing properties and, on activation, produces IL-22, TNF-α, IL-8 and IL-2, and activates endothelial cells. Tumour NCR + ILC3 may interact with both lung tumour cells and tumour-associated fibroblasts, resulting in the release of cytokines primarily on engagement of the NKp44-activating receptor. In patients, NCR + ILC3 are present in significantly higher amounts in stage I/II NSCLC than in more advanced tumour stages and their presence correlate with the density of intratumoral TLSs. Our results indicate that NCR + ILC3 accumulate in human NSCLC tissue and might contribute to the formation of protective tumour-associated TLSs. Innate lymphoid cells (ILCs) are emerging as a family of cells involved in innate anti-microbial immunity, tissue remodelling, lymphoid organogenesis and inflammation, in particular at barrier surfaces [1] , [2] . Natural killer (NK) cells, the first ILC discovered and the most widely distributed in different tissues, are regulated through a variety of activating and inhibitory cell surface receptors [3] , [4] , [5] . Current data are compatible with the concept that the ligands for activating NK receptors are expressed primarily by ‘stressed’ cells (including tumour or virus-infected cells). NKp46 (ref. 6 ), NKp30 (ref. 7 ) and NKp44 (ref. 8 ) are activating receptors (collectively named ‘natural cytotoxicity receptors’ (NCRs)) that play a major role in tumour cell recognition and killing by NK cells [9] . Although NCRs were found to bind some viral glycoproteins, their ligands on tumour cells have only partially been defined [10] , [11] . B7-H6 and, very recently, a novel isoform of the mixed-lineage leukemia (MLL5) protein have been shown to be expressed on a large panel of tumour cells [12] , [13] and are recognized by NKp30 and NKp44 receptors, respectively. Although a role of NK cells in anti-tumour immunity has been established, such a role for other ILC populations remains largely unexplored. Recently, three subsets of ILC have been identified on the basis of their cytokine expression patterns and dependency on transcription factors [14] , [15] , [16] , [17] . Notably, ILC subpopulations produce an array of cytokines that in variety match those of T-helper cell subsets. Besides conventional NK (cNK) cells, an additional ILC population expressing NCRs, but functionally different from NK cells, has been identified in both humans [18] , [19] , [20] , [21] , [22] and mice [23] , [24] , [25] . Unlike NK cells, in humans this NCR + cell population is dependent on the orphan nuclear receptor (ROR)γt transcription factor and on the interleukin (IL)-7Rα for its development and function. In addition, these cells constitutively express NKp44 but not CD94, lack perforin, granzymes and death receptors, while they produce IL-22 following cell activation [25] . These cells were termed NCR + ILC3, to identify a subgroup of human ILC3 distinct from lymphoid tissue inducer (LTi) cells [26] . Fate-mapping approaches showed that these cells are developmentally distinct from cNK cells and localize primarily in mucosal tissues [27] , [28] , in particular in the intestinal tract, where they are involved in regulation of epithelial homeostasis, immunity to extracellular bacteria and wound healing [14] , [18] , [29] , [30] . Notably, post-natal CD56 + RORγt + CD127 + cells from human tonsils have been shown to express high levels of NKp44 and NKp46 (ref. 31 ), to produce lymphotoxin-α and to exert LT-inducing ability, at least in vitro [19] , [31] . In different pathological conditions, T, B and dendritic cells (DCs) may be organized in structures termed tertiary lymphoid structures (TLSs) containing functional T- and B-cell zones. Such lymphoid tissue neogenesis shares molecular determinants with secondary lymphoid organ (SLO) ontogeny, including the release of LTα1β2 and tumour necrosis factor (TNF), and the expression, on stromal cells, of their respective receptors (LTβR and TNF receptor (TNFR)) [32] , [33] . These molecular interactions play a crucial role in the regulation of lymphocyte homing and compartmentalization, in both SLOs and TLSs, by inducing the expression of chemokines and adhesion molecules [34] , [35] . In mice, during the early stages of SLO development, membrane-bound LTα1β2 is expressed by fetal CD3 neg CD4 + CD45 + LTi cells [36] ; however, no clear evidence has been obtained that the adult counterparts of LTi cells (or ILCs with LTi activity) may orchestrate TLS formation or be recruited into inflamed tissues. Adult bronchus-associated lymphoid neogenesis is now recognized as a common feature of many chronic inflammatory diseases of the lung, such as tuberculosis [37] and chronic obstructive pulmonary disease [38] , and its formation is apparently independent from LTi cells [39] . However, limited information exists on lymphoid neogenesis in cancer, where it remains to be clarified whether TLS formation may represent a beneficial or, rather, a harmful event during cancer progression. In the case of human non-small cell lung cancer (NSCLC), it has been shown that TLSs are associated with a favourable prognosis, suggesting that they may participate in antitumoral immunity [40] . On the other hand, their formation could also represent a detrimental event, as suggested by a murine model of melanoma [41] . Therefore, it is important to clarify whether ILCs are present in tumours, in particular in humans, to define their functional capabilities and their possible involvement in tertiary lymphoid organ neogenesis. Here we identified NCR + ILC3-infiltrating human NSCLC. These cells produced proinflammatory cytokines and chemotactic factors on interaction with tumour cells or tumour-associated (TA) fibroblasts. Remarkably, tumour-infiltrating NCR + ILC3 accumulated at the edge of TA lymphoid aggregates and were endowed not only with proinflammatory but also with LTi functional capability. NCR + ILC3 accumulate in NSCLC tissues We have previously shown that a CD3 neg CD56 + NKp44 + cell population selectively infiltrates NSCLC, whereas it is virtually undetectable in normal lung tissues [42] . In addition, NCR + cells are mainly localized in the tumour stroma, in particular within stromal regions characterized by high density of lymphocytes [42] . As NCR + ILC3 express high levels of NKp44, these data prompted us to further investigate whether the various ILC subsets, and in particular Group 3 ILC expressing NCRs, were present in the tumour microenvironment. To this end, we employed a more stringent gating strategy, as shown in Fig. 1a , which allowed us to assess the frequency of the different ILC subsets in NSCLC tissue as well as in matched normal lung tissue and in peripheral blood (PB) of the same patient. To better characterize the presence of NCR + ILC3, NCR neg ILC3 and ILC1 among CD127 + ILC, we further analysed NKp44 + CD117 + cells for the expression of suitable markers (that is, RORγt, CCR6 and CD25). On the other hand, for the characterization of the different subsets of CD127 neg, ILCs, NKp44, NKp46, CD103 and T-bet were analysed. As expected, all CD127 neg NKp46 + ILCs expressed the transcription factor T-bet and, interestingly, the majority of NKp46 + NKp44 + cells expressed CD103, thus resembling the newly described intraepithelial ILC1 (ref 22 and Fig. 1b ). 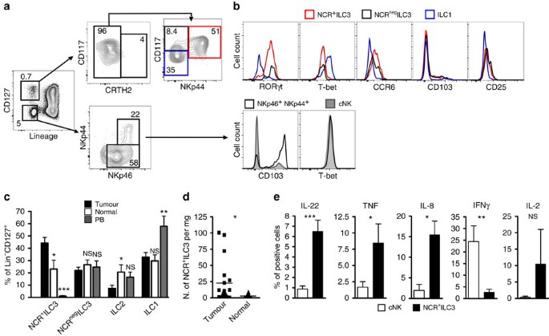Figure 1: Identification of CD127+ILC subsets in human NSCLC tissues. (a) MNCs isolated from NSCLC specimens were stained for CD3, CD14, CD19, CD34, BDCA2, CD80 (Lineage) and CD127, CRTH2, CD117, NKp46, NKp44, then gated on either Linneg/CD127+or Linneg/CD127negcells, as depicted. Among LinnegCD127+, ILC2 were identified as CRTH2+cells, NCRnegILC3 were identified as CD117+NKp44negcells (black), NCR+ILC3 were identified as CD117+NKp44+cells (red) and ILC1 were identified as CD117negNKp44negcells (blue). Among LinnegCD127negcells, cNK cells are here identified as NKp46+NKp44neg. Numbers in gates (outlined areas) indicate the percentage of cells in total viable CD45+MNC. One representative experiment is shown. (b) Flow cytometric analysis of the expression of surface and intranuclear markers in NSCLC CD127+ILC subsets and CD127negNKp46+subsets. One representative experiment out of 10 is shown. (c) Frequency ±s.e.m. of the various CD127+ILC populations in NSCLC (n=16) compared with matched normal lung tissues (n=10) and PB (n=7); NS, not significant; *P=<0.05, **P=<0.01, ***P=<0.001. Student’st-test. (d) Absolute number of NCR+ILC3 cells per mg of tissue in either neoplastic (n=16) or matched normal (n=10) lung tissues. *P=<0.05, Student’st-test. (e) Expression of IL-22, TNF, IL-8, IFNγ and IL-2 assessed in freshly isolated tumour NCR+ILC3 and tumour cNK cells stimulated for 6 h with PMA/ionomycin plus IL-23, and identified using the gating strategy shown ina. Graphs represent data from three to ten independent experiments; NS, not significant; *P=<0.05, **P=<0.01, ***P=<0.001 Student’st-test. Figure 1: Identification of CD127 + ILC subsets in human NSCLC tissues. ( a ) MNCs isolated from NSCLC specimens were stained for CD3, CD14, CD19, CD34, BDCA2, CD80 (Lineage) and CD127, CRTH2, CD117, NKp46, NKp44, then gated on either Lin neg /CD127 + or Lin neg /CD127 neg cells, as depicted. Among Lin neg CD127 + , ILC2 were identified as CRTH2 + cells, NCR neg ILC3 were identified as CD117 + NKp44 neg cells (black), NCR + ILC3 were identified as CD117 + NKp44 + cells (red) and ILC1 were identified as CD117 neg NKp44 neg cells (blue). Among Lin neg CD127 neg cells, cNK cells are here identified as NKp46 + NKp44 neg . Numbers in gates (outlined areas) indicate the percentage of cells in total viable CD45 + MNC. One representative experiment is shown. ( b ) Flow cytometric analysis of the expression of surface and intranuclear markers in NSCLC CD127 + ILC subsets and CD127 neg NKp46 + subsets. One representative experiment out of 10 is shown. ( c ) Frequency ±s.e.m. of the various CD127 + ILC populations in NSCLC ( n =16) compared with matched normal lung tissues ( n =10) and PB ( n =7); NS, not significant; * P =<0.05, ** P =<0.01, *** P =<0.001. Student’s t -test. ( d ) Absolute number of NCR + ILC3 cells per mg of tissue in either neoplastic ( n =16) or matched normal ( n =10) lung tissues. * P =<0.05, Student’s t -test. ( e ) Expression of IL-22, TNF, IL-8, IFNγ and IL-2 assessed in freshly isolated tumour NCR + ILC3 and tumour cNK cells stimulated for 6 h with PMA/ionomycin plus IL-23, and identified using the gating strategy shown in a . Graphs represent data from three to ten independent experiments; NS, not significant; * P =<0.05, ** P =<0.01, *** P =<0.001 Student’s t -test. Full size image As a whole, ILC composition in NSCLC tissues deeply differed from that in matched normal tissues and in patient PB ( Fig. 1c ). Among total Lineage neg CD127 + lymphoid cells, the frequency of NCR + ILC3 was significantly higher in tumour tissues (44.3%±4.5 of total CD127 + cells) than in matched normal lung (23%±7.2) or than in PB, where they were virtually absent (1%±0.5). No substantial difference in the frequency of NCR neg ILC3 was observed between NSCLC and the normal counterpart or lung cancer patient PB. On the contrary, tumour-infiltrating ILC2 were present in significantly lower amount (7.3%±2.6) if compared with normal tissues (20.6%±5.9). ILC1, which were mainly represented in patient PB, were present in similar amount in tumour and normal lung tissues. Thus, a specific accumulation of NCR + ILC3 occurs during the development of NSCLC. The preferential accumulation of NCR + ILC3 in tumour was more evident when their absolute number per mg of tissue was calculated (22.8±7.7 cells per mg in the tumour versus 2.9±1 cells per mg in the normal lung) ( Fig. 1d ). These data demonstrate that human NSCLC are infiltrated by a substantial amount of NCR + ILC3, otherwise sparsely represented in adjacent healthy lung tissues. NSCLC NCR + ILC3 are an abundant innate source of cytokines A specific feature of NCR + ILC3 is the production of IL-22 on IL-23 stimulation [18] . We therefore stimulated, NCR + ILC3 freshly isolated from NSCLC tissues with phorbol myristate acetate (PMA)/ionomycin and/or IL-23, and the production of the distinctive pattern of cytokines (IL-22, TNF, IL-8 and IL-2) was detected by intracytoplamic staining ( Fig. 1e and Supplementary Fig. 1a ), thus mirroring cytokines produced on the same stimulation by tonsil NCR + ILC3. However, a lower amount of IL-22 was released by tumour ILCs in comparison with the tonsillar counterpart ( Supplementary Fig. 1b ). To complete their functional characterization, tumour NCR + ILC3 were expanded in vitro . As a control, NCR + ILC3 were also isolated from human tonsils and cultured. Thus, NKp44 + CD127 + CD117 + cells were purified by flow cytometry cell sorting and cultured for 4–6 weeks in the presence of IL-2 and IL-7. On in - vitro proliferation, cells maintained all the hallmarks of NCR + ILC3. When compared with cultured cNK cells, they expressed high levels of CD117, CCR6, CXCR5 and CD25, and higher levels of NKp44 and CD161. In addition, they stably expressed RORγt, while surface NKp30 and NKp46 were expressed at lower levels than cNK cells. On the other hand, tumour-infiltrating NCR + ILC3 lacked typical cNK cell markers such as CD94, KIR and Perforin ( Fig. 2a ). 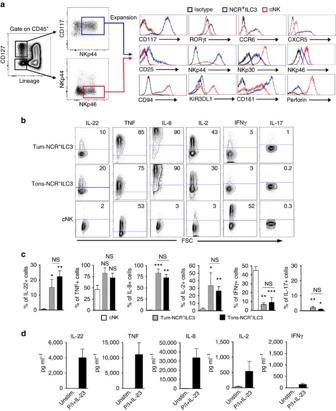Figure 2: Phenotype and cytokine expression profile of tumour NCR+ILC3. (a) Sorting strategy of NCR+ILC3 and cNK cells from lung tumour tissues according to the expression of CD117, NKp44 and NKp46 after gating on CD45+LinnegCD127+or LinnegCD127negcells (left panel). Lineage=(CD3/CD14/CD19/CD34/BDCA2/CD80/CRTH2). After sorting, both cNK and NCR+ILC3 were expandedin vitrofor 4–6 weeks and the specified phenotypic markers were assessed by flow cytometry (right panel). (b) Intracellular cytokine analysis of expanded tumour and tonsil NCR+ILC3 and cNK cells, stimulated for 6 h with PMA/ionomycin plus IL-23. One representative experiment out of eight is shown. Data of the eight experiments performed are summarized inc; bars represent the mean values of the percentage of positive cells±s.e.m. for the indicated cell population. *P=<0.05, **P<0.01 and ***P<0.005. (Student’st-test). (d) Cytokine detection in culture supernatants of tumour NCR+ILC3 (105cells per 200 μl) stimulated for 24 h with PMA/ionomycin plus IL-23. Bars represent mean values±s.e.m. of four to six independent experiments with tumour NCR+ILC3 from different patients. Figure 2: Phenotype and cytokine expression profile of tumour NCR + ILC3. ( a ) Sorting strategy of NCR + ILC3 and cNK cells from lung tumour tissues according to the expression of CD117, NKp44 and NKp46 after gating on CD45 + Lin neg CD127 + or Lin neg CD127 neg cells (left panel). Lineage=(CD3/CD14/CD19/CD34/BDCA2/CD80/CRTH2). After sorting, both cNK and NCR + ILC3 were expanded in vitro for 4–6 weeks and the specified phenotypic markers were assessed by flow cytometry (right panel). ( b ) Intracellular cytokine analysis of expanded tumour and tonsil NCR + ILC3 and cNK cells, stimulated for 6 h with PMA/ionomycin plus IL-23. One representative experiment out of eight is shown. Data of the eight experiments performed are summarized in c ; bars represent the mean values of the percentage of positive cells±s.e.m. for the indicated cell population. * P =<0.05, ** P <0.01 and *** P <0.005. (Student’s t -test). ( d ) Cytokine detection in culture supernatants of tumour NCR + ILC3 (10 5 cells per 200 μl) stimulated for 24 h with PMA/ionomycin plus IL-23. Bars represent mean values±s.e.m. of four to six independent experiments with tumour NCR + ILC3 from different patients. Full size image On stimulation, the cytokine expression profile was comparable to that of tonsil NCR + ILC3, while it was markedly distinct from that of cNK cells ( Fig. 2b,c ). Both tumour and tonsil NCR + ILC3 produced significant amount of IL-22, TNF-α, IL-8 and IL-2 on stimulation. On the contrary, differently from cNK cells, IFNγ production could barely be detected, whereas IL-17 was not produced by any of the ILC subsets analysed ( Fig. 2b,c ). To quantify the amount of cytokines released by tumour NCR + ILC3, the production of relevant cytokines was also confirmed by assessing their presence in culture supernatants on stimulation by PMA/ionomycin and IL-23 ( Fig. 2d ). In addition, tumour-infiltrating NCR + ILC3 did not produce IL-13, IL-5, IL-4 and IL-10 (data not shown). It is noteworthy that the same cytokine pattern was detectable in NCR + ILC3 freshly isolated from cancer specimens ( Fig. 1e ), thus confirming that tumour-infiltrating NCR + ILC3 maintain a stable phenotype after their ex - vivo culture and expansion in the presence of IL-7 and IL-2. Taken together, these findings suggest that NCR + ILC3 may play a role in tumour microenvironment because of the release of proinflammatory cytokines (TNF-α and IL-22) and by providing an innate source of cytokines mediating leukocyte recruitment and growth, such as IL-8 and IL-2, respectively. NCR + ILC3 recognize lung tumor cells via NKp44 The cellular ligands of NCRs are mainly expressed by abnormal cells such as infected or neoplastic cells [10] , [43] . Therefore, we investigated whether NCR + ILC3 present in lung tumours could interact with lung tumour cells via their surface NCRs. To this end, we employed a series of human NSCLC cell lines (both adenocarcinoma and squamous cell carcinoma) expressing NCR ligands ( Supplementary Fig. 2 ). First, we assessed whether NCR + ILC3 could exert any cytotoxic activity against lung tumour cells. No substantial cytolytic activity against NSCLC cells could be detected even at high effector/target (E/T) ratios, as predictable by the absence of lytic granules ( Fig. 2a ). Conversely, cNK cells efficiently lysed the same target cells ( Fig. 3a ). 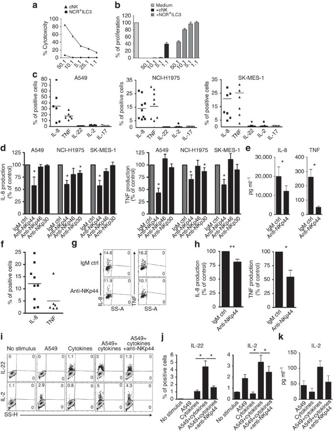Figure 3: Interactions between tumour NCR+ILC3 and NSCLC cells. (a) Cytotoxic activity of tumour NCR+ILC3 and cNK cells against A549 cells, at the indicated effector/target ratios, determined by a standard51Cr release assay. (b) Percentage of proliferation of A549 cells cultured for 4 days alone or in the presence of different amounts of either tumour NCR+ILC3 or cNK cells. (c) Intracellular cytokine expression of tumour NCR+ILC3 in the presence of three different lung tumour cell lines (A549, NCI-H1975 and SK-MES-1) on a 6 h co-culture period; E/T ratio=1:1. (d) Intracellular IL-8 and TNF expression by NCR+ILC3 following stimulation with the three different lung tumour cells was assessed in the presence of blocking monoclonal antibodies (mAbs) against the various NCRs (black columns) or isotypic control (grey column); E/T ratio=1:1. Data shown represent mean values±s.e.m. of the results obtained from five to nine independent experiments. *P≤0.05, Wilcoxon signed-rank test. (e) IL-8 and TNF release in culture supernatants of tumour NCR+ILC3 following stimulation with A549 tumour cells (105cells; E/T ratio: 1:1), for 24 h, in the presence of blocking mAbs against NKp44 or isotypic control. Data represent mean values±s.e.m. of the results obtained from six independent experiments. *P≤0.05, Student’st-test. (f) IL-8 and TNF production by freshly isolated tumour NCR+ILC3 following stimulation with A549 lung tumour cells on a 6-h co-culture period. Freshly isolated NCR+ILC3 were identified as inFig. 1a. E/T ratio=1 CD45+mononuclear cells: 1 target cell. (g) IL-8 and TNF expression by freshly isolated tumour NCR+ILC3 stimulated with A549 cells in the presence or absence of a blocking mAb against the NKp44 receptor. Data obtained in nine (IL-8) and six (TNF) independent experiments are summarized inh. Bars represent mean values±s.e.m. of the results obtained for the indicated cytokines. *P≤0.05, **P≤0.01, Student’st-test. (i) IL-22 and IL-2 production by NCR+ILC3 stimulated as indicated. Cytokines indicates a mixture of IL-1β+IL-7+IL-23. Data obtained from five independent experiments are summarized inj. Bars represent mean values±s.e.m. of the results obtained for the indicated cytokines. *P≤0.05, Student’st-test. Release of relevant cytokines by tumour NCR+ILC3 (105cells per 200 μl) under the same stimulatory conditions was also confirmed by analysing culture supernatants (k). Bars represent mean values±s.e.m. of data obtained from six to eight experiments. Figure 3: Interactions between tumour NCR + ILC3 and NSCLC cells. ( a ) Cytotoxic activity of tumour NCR + ILC3 and cNK cells against A549 cells, at the indicated effector/target ratios, determined by a standard 51 Cr release assay. ( b ) Percentage of proliferation of A549 cells cultured for 4 days alone or in the presence of different amounts of either tumour NCR + ILC3 or cNK cells. ( c ) Intracellular cytokine expression of tumour NCR + ILC3 in the presence of three different lung tumour cell lines (A549, NCI-H1975 and SK-MES-1) on a 6 h co-culture period; E/T ratio=1:1. ( d ) Intracellular IL-8 and TNF expression by NCR + ILC3 following stimulation with the three different lung tumour cells was assessed in the presence of blocking monoclonal antibodies (mAbs) against the various NCRs (black columns) or isotypic control (grey column); E/T ratio=1:1. Data shown represent mean values±s.e.m. of the results obtained from five to nine independent experiments. * P ≤0.05, Wilcoxon signed-rank test. ( e ) IL-8 and TNF release in culture supernatants of tumour NCR + ILC3 following stimulation with A549 tumour cells (10 5 cells; E/T ratio: 1:1), for 24 h, in the presence of blocking mAbs against NKp44 or isotypic control. Data represent mean values±s.e.m. of the results obtained from six independent experiments. * P ≤0.05, Student’s t -test. ( f ) IL-8 and TNF production by freshly isolated tumour NCR + ILC3 following stimulation with A549 lung tumour cells on a 6-h co-culture period. Freshly isolated NCR + ILC3 were identified as in Fig. 1a . E/T ratio=1 CD45 + mononuclear cells: 1 target cell. ( g ) IL-8 and TNF expression by freshly isolated tumour NCR + ILC3 stimulated with A549 cells in the presence or absence of a blocking mAb against the NKp44 receptor. Data obtained in nine (IL-8) and six (TNF) independent experiments are summarized in h . Bars represent mean values±s.e.m. of the results obtained for the indicated cytokines. * P ≤0.05, ** P ≤0.01, Student’s t -test. ( i ) IL-22 and IL-2 production by NCR + ILC3 stimulated as indicated. Cytokines indicates a mixture of IL-1β+IL-7+IL-23. Data obtained from five independent experiments are summarized in j . Bars represent mean values±s.e.m. of the results obtained for the indicated cytokines. * P ≤0.05, Student’s t -test. Release of relevant cytokines by tumour NCR + ILC3 (10 5 cells per 200 μl) under the same stimulatory conditions was also confirmed by analysing culture supernatants ( k ). Bars represent mean values±s.e.m. of data obtained from six to eight experiments. Full size image Next, we assessed whether TA NCR + ILC3 could inhibit tumour cell growth in co-culture experiments. Also in this case, virtually no inhibition could be detected in a 4-day proliferation assay. Only a marginal inhibition was observed at 50:1 ratio ( Fig. 3b ). Although NCR + ILC3 did not show any cytolytic and tumour-growth suppressing abilities, they were able to efficiently recognize lung tumour cells as revealed by cytokine production after co-culture with a variety of lung tumour cell lines (A549, NCI-H1975 and SK-MES1) ( Fig. 3c ). Recognition of NSCLC cells by tumour NCR + ILC3 resulted in a strong production of TNF and IL-8 but very low level of IL-2 and IL-22. The production of IL-17 was never detectable. As control, epithelial cells from normal lung (isolated as described in Methods section) were also employed as target cells and, as expected, no cytokine production by tumour NCR + ILC3 was observed. It has recently been reported that the engagement of NKp44 in RORγt + ILC can trigger a coordinated proinflammatory programme [30] . Therefore, we investigated whether NCRs could be involved in the cytokine production induced by the interaction between NCR + ILC3 and lung tumour cells. Thus, cytokine production was analysed on NCR + ILC3 exposure to lung tumour cells in the presence or in the absence of blocking monoclonal antibodies specific for NKp44, NKp46 and NKp30. In line with the differences in the levels of expression of NKp30, NKp46 and NKp44 ( Fig. 2a ), NKp44 receptor appeared as the most involved NCR during interactions with the different cancer cell lines. Remarkably, blocking of NKp44 receptor caused a marked and consistent decrease in the production of TNF-α and IL-8, whereas blocking of other NCRs resulted in a marginal inhibition of cytokine production ( Fig. 3d ). These data were confirmed by also assessing the amount of cytokines released in the culture supernatants ( Fig. 3e ). Interestingly, we confirmed the effect of blocking NKp44 also on freshly isolated NCR + ILC3, as both IL-8 and TNF production was significantly inhibited by blocking the NKp44 receptor ( Fig. 3f–h ). Despite stimulation of tumour NCR + ILC3 by NSCLC cells resulted in low production of IL-2 and IL-22, we observed that the recognition of cancer cells by NKp44 strongly increased the production of IL-2 and IL-22 induced by the proinflammatory cytokines IL-1β and IL-23 ( Fig. 3i–k ). These data clearly indicate that tumour NCR + ILC3 can efficiently recognize cancer cells, and that NKp44 plays a relevant role in this interaction. Of note, the strength of NKp44-mediated triggering of NCR + ILC3 was not due to a higher expression of the NKp44 ligand(s) on NSCLC cells employed as cell target. Indeed, the three NCR ligands were similarly involved in the recognition of NSCLC cells by cNK cells, with NKp46 ligand actually playing a major role ( Supplementary Fig. 2 ), thus ruling out a preferential expression of NKp44 ligand(s) on target cells. NCR + ILC3 produce IL-8 upon interaction with TA fibroblasts Fibroblasts are an important component of the tumour microenvironment. They have recently been reported to exert a strong immunosuppressive activity on cNK cells [44] . Therefore, we further analysed the effect of the interactions between NCR + ILC3 and lung TA fibroblasts. Remarkably, NCR + ILC3 efficiently recognized TA fibroblasts, as this interaction led to the production of TNF-α and IL-8 but not of IL-22 ( Fig. 4a ). Interestingly, the production of IL-8 was consistently higher than TNF-α, observed as both intracytoplasmic staining ( Fig. 4a ) and cytokine content in the culture supernatants ( Fig. 4d ). As we noticed that TA fibroblasts expressed the ligands for NKp44 and, partially, NKp30 ( Fig. 4b ), we analysed whether these NCRs were involved in the interaction between tumour-infiltrating NCR + ILC3 and TA fibroblasts. Antibody-mediated blocking of NKp44 strongly inhibited the production and the release of TNF-α but not IL-8 ( Fig. 4c,d ). On the contrary, blocking of NKp30 and NKp46 had no inhibitory effect. 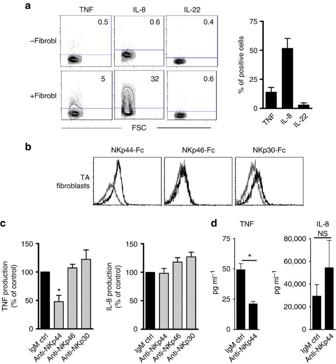Figure 4: Triggering of intratumoral NCR+ILC3 by TA fibroblasts. Intracellular cytokine analysis of tumour NCR+ILC3 in the absence or in the presence of TA fibroblasts during a 6-h co-culture period. Numbers in quadrants indicate positive cells in each (left); E/T ratio=1:1. Data obtained in eight independent experiments are summarized in the right panel ofa. Bars represent mean values±s.e.m. of the results obtained for the indicated cytokines. (b) Staining of TA fibroblasts with soluble NKp44Fc, NKp46Fc, NKp30Fc receptors (black line) or isotype control (grey line). (c) Intracellular cytokine production by NCR+ILC3 cultured with TA fibroblasts for 6 h (E/T ratio: 1:1) was assessed in the presence of blocking monoclonal antibodies (mAbs) against NCRs (grey columns) or isotypic control (black column). Data shown represent mean values±s.e.m. of the results obtained from five to nine independent experiments. *P≤0.05, Wilcoxon signed-rank test. (d) Cytokine release in culture supernatants by tumour NCR+ILC3 (105cells per 200 μl) co-cultured with TA fibroblasts for 24 h (E/T ratio: 1:1) in the presence of blocking mAbs against NKp44 or isotypic control. Data shown represent mean values±s.e.m. of the results obtained from six experiments. *P≤0.05. Figure 4: Triggering of intratumoral NCR + ILC3 by TA fibroblasts. Intracellular cytokine analysis of tumour NCR + ILC3 in the absence or in the presence of TA fibroblasts during a 6-h co-culture period. Numbers in quadrants indicate positive cells in each (left); E/T ratio=1:1. Data obtained in eight independent experiments are summarized in the right panel of a . Bars represent mean values±s.e.m. of the results obtained for the indicated cytokines. ( b ) Staining of TA fibroblasts with soluble NKp44Fc, NKp46Fc, NKp30Fc receptors (black line) or isotype control (grey line). ( c ) Intracellular cytokine production by NCR + ILC3 cultured with TA fibroblasts for 6 h (E/T ratio: 1:1) was assessed in the presence of blocking monoclonal antibodies (mAbs) against NCRs (grey columns) or isotypic control (black column). Data shown represent mean values±s.e.m. of the results obtained from five to nine independent experiments. * P ≤0.05, Wilcoxon signed-rank test. ( d ) Cytokine release in culture supernatants by tumour NCR + ILC3 (10 5 cells per 200 μl) co-cultured with TA fibroblasts for 24 h (E/T ratio: 1:1) in the presence of blocking mAbs against NKp44 or isotypic control. Data shown represent mean values±s.e.m. of the results obtained from six experiments. * P ≤0.05. Full size image Overall, these results indicate that NCR + ILC3 might actively interact with fibroblasts present in the tumour microenvironment, leading to the release of high amounts of leukocyte chemotactic factors. At the same time, they release proinflammatory cytokines such as TNF-α influencing the vascular permeability and acting on other neighbouring cell types of both haematopoietic and non-haematopoietic origin. Tumor NCR + ILC3 display LTi potential and associate with TLS The prototypical group 3 ILC are LTi cells, which are crucial for the formation of SLOs during embryogenesis. Although this ILC subset lacks NCRs and can distinctively produce IL-17A, it shares many development and functional features with NCR + ILC3, which justify their joint subgrouping as ILC3. Therefore, we hypothesized that NCR + ILC3 isolated from NSCLC might show LT-inducing properties. It has previously been reported that Lin neg NKp44 + CD127 + cells (both CD56 + and CD56 neg ) induce the expression of vascular cell adhesion molecule-1 (VCAM-1) and intercellular adhesion molecule 1 (ICAM-1) on mesenchymal stem cells (MSCs) when co-cultured for 4 days in the presence of IL-7. This functional property has been regarded as a marker of the LT-inducing ability mainly due to the production of specific molecules such as TNFα and lymphotoxins (LTα1β2 or LTα3) [19] , [31] . Therefore, we assessed whether tumour-infiltrating NCR + ILC3 had this property as well. NCR + ILC3 isolated from tonsils were used as a positive control. As shown in Fig. 5a , lung cancer-derived NCR + ILC3 induced a significant upregulation of the adhesion molecules ICAM-1 and VCAM-1 on MSCs. 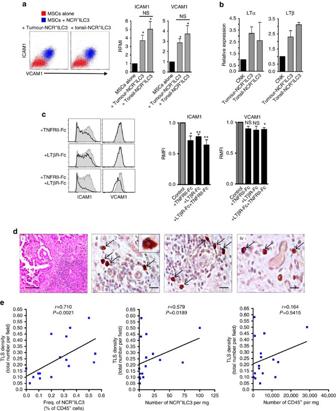Figure 5: Lymphoid tissue-inducing properties of tumour-derived NCR+ILC3. (a) Expression of ICAM-1 and VCAM-1 on MSCs cultured for 4 days alone or with tumour or tonsil NCR+ILC3. One representative experiment out of nine is shown (left panels). Relative mean fluorescent intensity (RFMI) of the expression of ICAM-1 and VCAM-1 by MSCs co-cultured without or with tumour or tonsil NCR+ILC3 (mean value±s.e.m.). *P≤0.05, Student’st-test. (b) LTα and LTβ mRNA was detected by quantitative reverse transcription–PCR in tumour or tonsil NCR+ILC3 and cNK cells. Bars represent mean fold change±s.e.m. relative to cNK cells of three independent experiments, after normalizing to glyceraldehyde 3-phosphate (GAPDH). (c) Expression of ICAM-1 and VCAM-1 on MSCs cultured with tumour NCR+ILC3 cells for 4 days in the presence of irrelevant Fc chimera (grey line) or soluble LTβR-Fc and/or TNFRII-Fc chimeras (black line). A representative experiment is shown in the left panels (histograms). Bars in the right panels represent mean±s.e.m. of RMFI obtained in six independent experiments. *P≤0.05, Student’st-test. (d) Lymphoid follicle-like structures and NKp46+RORγt+cells in human NSCLC. Lymphoid follicle-like structures are frequently observed in the stromal compartment of NSCLC (i). NKp46+(brown)RORγt+(red) double positive lymphoid cells (arrows) located at the edge of small lymphoid aggregates (ii and iii) or nearby small blood vessels (iv). The insert in ii shows a magnification of a double positive cell. (i): × 200; (ii,iii,iv): × 630; insert: × 1,000. Scale bars, 50 μm (i) and 20 μm (ii, iii,iv). (e) Correlation between the density of TLS and the frequency of NCR+ILC3 among tumour-infiltrating CD45+cells (left panel), the absolute number of NCR+ILC3 per mg of neoplastic tissue (middle panel) and the absolute number of total CD45+cells per mg of neoplastic tissue (right panel) (linear regression test). Figure 5: Lymphoid tissue-inducing properties of tumour-derived NCR + ILC3. ( a ) Expression of ICAM-1 and VCAM-1 on MSCs cultured for 4 days alone or with tumour or tonsil NCR + ILC3. One representative experiment out of nine is shown (left panels). Relative mean fluorescent intensity (RFMI) of the expression of ICAM-1 and VCAM-1 by MSCs co-cultured without or with tumour or tonsil NCR + ILC3 (mean value±s.e.m.). * P ≤0.05, Student’s t -test. ( b ) LTα and LTβ mRNA was detected by quantitative reverse transcription–PCR in tumour or tonsil NCR + ILC3 and cNK cells. Bars represent mean fold change±s.e.m. relative to cNK cells of three independent experiments, after normalizing to glyceraldehyde 3-phosphate (GAPDH). ( c ) Expression of ICAM-1 and VCAM-1 on MSCs cultured with tumour NCR + ILC3 cells for 4 days in the presence of irrelevant Fc chimera (grey line) or soluble LTβR-Fc and/or TNFRII-Fc chimeras (black line). A representative experiment is shown in the left panels (histograms). Bars in the right panels represent mean±s.e.m. of RMFI obtained in six independent experiments. * P ≤0.05, Student’s t -test. ( d ) Lymphoid follicle-like structures and NKp46 + RORγt + cells in human NSCLC. Lymphoid follicle-like structures are frequently observed in the stromal compartment of NSCLC (i). NKp46 + (brown)RORγt + (red) double positive lymphoid cells (arrows) located at the edge of small lymphoid aggregates (ii and iii) or nearby small blood vessels (iv). The insert in ii shows a magnification of a double positive cell. (i): × 200; (ii,iii,iv): × 630; insert: × 1,000. Scale bars, 50 μm (i) and 20 μm (ii, iii,iv). ( e ) Correlation between the density of TLS and the frequency of NCR + ILC3 among tumour-infiltrating CD45 + cells (left panel), the absolute number of NCR + ILC3 per mg of neoplastic tissue (middle panel) and the absolute number of total CD45 + cells per mg of neoplastic tissue (right panel) (linear regression test). Full size image The expression of lymphotoxins α and β is considered another relevant LTi property that has previously been detected in human tonsil NCR + ILC3 (ref. 19 ). We found that NCR + ILC3 isolated from lung cancers expressed lymphotoxins messenger RNA at levels comparable to those of the tonsil counterpart ( Fig. 5b ). Because of these latter data and of evidence of an abundant TNFα production by tumour NCR + ILC3, we investigated the role of these factors in the upregulation of adhesion molecules on MSCs. LTα1β2 binds LTβ receptor (LTβR) on MSCs, whereas TNFα and LTα3 share the TNFRII. Thus, by preventing the engagement of these factors on their receptors using TNFRII- and LTβR-soluble molecules, individually or in combination, we assessed their role in the upregulation of adhesion molecules on MSCs. Both pathways appeared involved and the synergistic effect of the two signals seems required for the upregulation of VCAM-1 ( Fig.5c ). In line with these findings on possible LTi properties of intratumoral NCR + ILC3, we observed that these cells were localized at the edge of lymphoid structures associated to NSCLC. Double staining of lung tissue sections with anti-NKp46 and anti-RORγt Abs revealed that in the normal lung tissue, in the peri-bronchial connective tissue, below the normal respiratory epithelium, NKp46 + RORγt + lymphoid cells were undetectable. In contrast, in lung adenocarcinomas, in which lymphoid-like follicles are usually detectable ( Fig. 5d (i) ), NKp46 + RORγt + cells were interspersed within the stromal compartment and were often localized at the edge of lymphoid aggregates ( Fig. 5d (ii,iii) ) or near small blood vessels ( Fig. 5d (iv) ) On the basis of their functional properties and of their location within tumour tissue, we analysed whether the presence of NSCLC-associated NCR + ILC3 could be related to the formation of ectopic lymphoid tissues. We found that both the percentage of NCR + ILC3 in total leukocytes (CD45 + cells) infiltrating the tumour and the absolute number of tumour NCR + ILC3 per mg of NSCLC tissue correlated with the density of TLSs in cancer tissues ( Fig. 5e ). This correlation was independent from the amount of leukocyte infiltrating the tumour, as the absolute number of tumour-infiltrating CD45 + cells did not correlate with TLSs. These results suggest that NCR + ILC3-infiltrating lung cancers are endowed with LTi properties and might contribute to the formation and/or maintenance of TLSs or lymphoid aggregates at the tumour site. ILC3 triggering via NCRs results in endothelium activation The recruitment of leukocytes from blood into peripheral tissues requires the passage of cells across the vascular endothelium. This process is tightly controlled and regulated by the expression of adhesion molecules on endothelial surfaces. As NCR + ILC3 produce large amounts of pro-inflammatory (TNF-α) and chemotactic/angiogenic factors (IL-8), we assessed the activating potential of these factors on endothelial cells. NCR + ILC3 were triggered using a mixture of anti-NKp44, NKp30 and NKp46 monoclonal antibodies and, after 24 h, the supernatants were collected and employed for functional assays on endothelial cells. Supernatants derived from NCR-triggered NCR + ILC3 acted on endothelial cells by strongly increasing their adhesive properties on gelatin-coated wells, as observed by a cell-adhesion test ( Fig. 6a ). The increased adherence of endothelial cells to extracellular matrix was accompanied by the upregulation of adhesion molecules involved in cell-to-cell adhesion, including a statistically significant upregulation of ICAM-1 and VCAM-1 ( Fig. 6b ), most probably secondary to TNF release. These results indicated that an innate activation of NCR + ILC3 might favour the recruitment of other leukocytes in tumour tissue. As NCR + ILC3 isolated from NSCLC produced high amount of IL-8, also known as neutrophil chemotactic factor, we investigated, whenever possible, whether the presence of intratumoral NCR + ILC3 might influence the recruitment of neutrophils. Although many other cells in the tumour microenvironment may represent a suitable source of IL-8, including macrophages, epithelial and endothelial cells, we found an interesting correlation between the amount of neutrophils and of NCR + ILC3-infiltrating NSCLC tissues ( Supplementary Fig. 3b ). 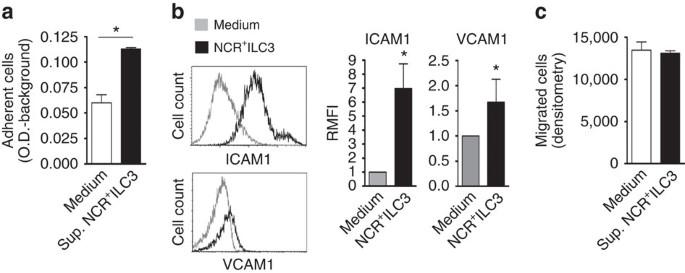Figure 6: Pro-inflammatory activity of tumour NCR+ILC3 on human endothelial cells. The adhesion capabilities and the migration of human umbilical vein endothelial cells (HUVEC cells) were analysed in the presence of conditioned medium derived from a NCR+ILC3 culture stimulated by a mixture of anti-NCR monoclonal antibodies (mAbs). (a) HUVEC cell adhesion on gelatin is doubled in the presence of conditioned medium of NCR+ILC3 stimulated by agonistic anti-NCRs mAbs as compared with unstimulated controls (each group,n=3) (mean value±s.e.m.). *P≤0.05, Student’st-test. (b) Expression of ICAM-1 and VCAM-1 on EAhy-926 cells co-cultured for 4 days alone or with tumour NCR+ILC3 at a ratio 1:1. One representative experiment out of nine is shown. Results obtained in nine independent experiments are summarized in the right panel. Data shown represent the relative mean fluorescent intensity (RFMI)±s.e.m. of the expression of ICAM-1 and VCAM-1 on EAhy-926 cells. *P≤0.05, Student’st-test. (c) HUVEC cell migration is not influenced by the presence of antibody-triggered NCR+ILC3 conditioned medium (each group,n=3). Figure 6: Pro-inflammatory activity of tumour NCR + ILC3 on human endothelial cells. The adhesion capabilities and the migration of human umbilical vein endothelial cells (HUVEC cells) were analysed in the presence of conditioned medium derived from a NCR + ILC3 culture stimulated by a mixture of anti-NCR monoclonal antibodies (mAbs). ( a ) HUVEC cell adhesion on gelatin is doubled in the presence of conditioned medium of NCR + ILC3 stimulated by agonistic anti-NCRs mAbs as compared with unstimulated controls (each group, n =3) (mean value±s.e.m.). * P ≤0.05, Student’s t -test. ( b ) Expression of ICAM-1 and VCAM-1 on EAhy-926 cells co-cultured for 4 days alone or with tumour NCR + ILC3 at a ratio 1:1. One representative experiment out of nine is shown. Results obtained in nine independent experiments are summarized in the right panel. Data shown represent the relative mean fluorescent intensity (RFMI)±s.e.m. of the expression of ICAM-1 and VCAM-1 on EAhy-926 cells. * P ≤0.05, Student’s t -test. ( c ) HUVEC cell migration is not influenced by the presence of antibody-triggered NCR + ILC3 conditioned medium (each group, n =3). Full size image On the other hand, IL-8 released by tumour NCR + ILC3 does not seem to be involved in angiogenetic processes. Supernatants derived from NCR-triggered NCR + ILC3 did not modify the basal migration of endothelial cells in vitro ( Fig. 6c ), thus suggesting that neo-angiogenesis would not represent a main consequence of TA NCR + ILC3 activation. Collectively, these findings indicate that NCR + ILC3 present in the lung tumour microenvironment may contribute to promote an inflammatory activation of the endothelium (see also their detection in close proximity of intratumoral blood vessels, Fig. 5d (iv) ). This would favour the recruitment of PB leukocytes and their infiltration and accumulation within the tumour mass. Frequency of tumour NCR + ILC3 decreases in advanced NSCLC As we found a correlation between the density of intratumoral TLS in NSCLC and the amount of NCR + ILC3 in the tumour infiltrate, and it has been reported that these TLSs correlate with higher survival rate [40] , we hypothesized that NCR + ILC3 might also be associated with a better tumour prognosis. A major prognostic factor for the survival of lung cancer patients is tumour stage [45] , [46] . Analyses of possible correlation between NCR + ILC3-infiltrating lung tumours and tumour stages revealed that samples from patients in stage I and stage II contained proportions of NCR + ILC3 significantly higher than those from patients in stage III (mean value 0.4%, and 0.41% versus 0.14% of CD45 + cells, respectively) ( Fig. 7 ). 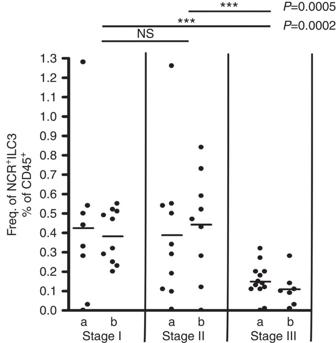Figure 7: Frequency of NCR+ILC3 in NSCLC tissues resected in patients with different stage of tumour disease. Data show the frequency of NCR+ILC3 among the total CD45+cell population isolated from 57 NSCLC of patients in stage I (18 patients; 8 in stage Ia and 10 in stage Ib), stage II (19 patients; 10 in stage IIa and 9 in stage IIb) and stage III (20 patients; 13 in stage IIIa and 7 in stage IIIb). Figure 7: Frequency of NCR + ILC3 in NSCLC tissues resected in patients with different stage of tumour disease. Data show the frequency of NCR + ILC3 among the total CD45 + cell population isolated from 57 NSCLC of patients in stage I (18 patients; 8 in stage Ia and 10 in stage Ib), stage II (19 patients; 10 in stage IIa and 9 in stage IIb) and stage III (20 patients; 13 in stage IIIa and 7 in stage IIIb). Full size image No significant differences in the amount of NCR + ILC3 were observed between cancer specimens of patients affected by adenocarcinomas or squamous cell carcinomas. In addition, smoking habit did not seem to influence NCR + ILC3 accumulation in cancer tissues. Thus, NCR + ILC3 are present in the microenvironment of NSCLC but are prone to disappear on disease progression. A low amount of NCR + ILC3 within NSCLC appears indeed associated with more advanced tumour stages and, therefore, potentially, with a poorer prognosis. Lung cancer is the most common cause of cancer-related mortality in the world. Over 80% of cases are represented by NSCLCs, which include adenocarcinomas and squamous cell carcinomas. In such tumours, the presence of TLS composed of mature DC/T-cell clusters and B-cell follicles has been widely documented [47] . Such structures have not been detected in sites distant from the tumour lesions, suggesting that they are likely to be formed in response to tumour cells and their microenvironment. Remarkably, it has recently been shown through univariate analysis that the density of TLS is predictive of survival in patients with early-stage NSCLC [40] . Our present results show that NCR + ILC3, a recently described subset of human innate lymphocytes, are present in lung tumours and may be involved in the production of a proinflammatory response in the tumour microenvironment. Analysis of their functional properties revealed that NCR + ILC3 may promote the recruitment of other leukocytes to the tumour site by secreting chemotactic factors and activating TA vessels. Of note, tumour NCR + ILC3 also display peculiar LTi properties and might therefore contribute to the formation and/or maintenance of tertiary lymphoid organs or lymphoid aggregates at the tumour site. In agreement with this hypothesis we found that the amount of NCR + ILC3 within tumour infiltrate correlated with the density of intratumoral TLS. Although other lymphocytes of the tumour microenvironment may produce a similar pattern of soluble factors, including LTα/β and TNF-α, which are critical for the possible LTi properties, NCR + ILC3 may play an exclusive role in the tumour microenvironment: first, they might be directly activated by cancer cells via NKp44 and therefore represent an early innate source of relevant cytokines; then compared with intratumoral NK cells, which may also be directly activated by cancer cells [42] , [48] , NCR + ILC3 apparently lack inhibitory receptors controlling their activities and can also provide a unique innate source of IL-2, a crucial growth factor for the clonal expansion of tumour-specific lymphocytes. On the other hand, the role of an innate source of IL-22 within tumour microenvironment remains to be identified and might even favour cancer cell growth [49] . Nevertheless, it is noteworthy that tumour NCR + ILC3 consistently released lower amount of IL-22 if compared with tonsillar counterpart ( Supplementary Fig. 1b ). Other relevant cytokines such as IL-8, TNFs, granulocyte–macrophage colony-stimulating factor [30] could also be released by NCR + ILC3 on the engagement of NKp44 by cancer cells, again providing critical factors for organizing the immune response. These latter soluble factors can also be released by other cells of the innate immunity, which, however, generally fail to be directly triggered by tumour cells. Tumour staging is the dominant prognostic factor for NSCLC patient survival [45] , [46] . Our data show that a higher frequency of NCR + ILC3 in NSCLC was associated with less advanced stages of NSCLC. Thus, the presence of NCR + ILC3, as for TLS [40] , [50] , could be related to a protective immunity and a more favourable tumour prognosis. Further studies, beyond the scope of the present contribution, are clearly required to better document this association and its putative prognostic value. The evidence of a reduced frequency of NCR + ILC3 in tumour samples of stage III patients raises the question of the reason of the disappearance of this lymphocyte subset. We could speculate that a more tolerogenic microenvironment is likely to operate in more advanced cancers, where the sustained release of inhibitory cytokines affect most immune cells. The maintenance and proliferation of ILC are promoted by common γ-chain cytokines such as IL-2, IL-7 and IL-15, which are mainly produced by haematopoietic cells (mainly myeloid and T cells) and, in part, by non-haematopoietic cells (stromal, endothelial and epithelial cells). Persistent inhibitory environmental signals within tumour tissue could therefore affect the presence of ILC via different pathways acting on different cells present in the tumour microenvironment. However, an active plasticity of ILC has lately been reported [51] and we favour the intriguing hypothesis that a more pronounced inflammation, occurring in later phases of tumour progression, could induce ILC3 to ILC1 transition. However, as the mere count of ILC1 versus ILC3 in tumour tissue would not obviously be sufficient to clarify this issue, further investigation will be required to corroborate this hypothesis. A tumour is composed of different cell types including malignant, stromal, endothelial and immune cells that form a heterogeneous network and exhibit complex interactions. The finding that ILC expressing NCRs may be present in the tumour tissues is particularly interesting. NCR ligands are highly expressed in tumours as revealed by the direct or indirect (that is, by the use of soluble NCR molecules) detection and by receptor masking-based cytolytic assays [9] . It has recently been reported that RORγt + ILC can sense and react to environmental signals via NCRs (independently of proinflammatory cytokines) [30] . Here we provide clear evidence that NCR + ILC3 present in the tumour tissues can be directly triggered by tumour cells, as well as by TA fibroblasts. This occurs mainly via the engagement of the NKp44 receptor, which is highly expressed by NCR + ILC3-infiltrating NSCLC. We observed an elevated production of both TNF-α and IL-8 on triggering of NKp44 by NSCLC cells. At the same time, as previously reported for tonsil and intestinal ILC3 (ref. 30 ), we observed a strong synergism for the secretion of IL-22 and IL-2 when TA NCR + ILC3 where activated by both NKp44 triggering and cytokines such as IL-1β and IL-23. On the other hand, in the case of the interaction with TA fibroblasts, blocking of NKp44 strongly inhibited TNF-α but not IL-8 production. These data suggest that in addition to NKp44, other cellular signals, still unidentified, may act on NCR + ILC3 for the fine-tuning of their cytokine production. Thus, activation of NCR + ILC3 is likely to occur within lung cancer tissues because of the abundant presence of NCR ligands on cells of the tumour microenvironment. The resulting cytokine release may induce leukocyte recruitment and proliferation (IL-8 and a unique innate source of human IL-2) [52] , [53] , inflammation (TNF-α) [54] and generation/maintenance of lymphoid tissues (LTα/β, TNF) [19] . Although it is still unclear whether intratumoral TLS represent simple lymphoid aggregates or functional immune structures, their association with a better survival probability suggests that the immune response to the tumour may be initiated in the tumour itself. In this context, it has been reported that extranodal lymphoid structures may participate in the induction of specific immune responses [55] , [56] . Considering that TLS contain high number of antigen-presenting DCs [40] , the possible occurrence of an intratumoral cancer-specific T-cell priming (in addition to the conventional priming occurring in SLO) could influence the evolution of the tumour and therefore the clinical outcome. tumour-associated antigens (TAAs) should be continuously sampled and stimulate specific T cells, increasing the efficiency and specificity of their priming. During tumour progression, TLS may allow T cells to react more rapidly to the shift in the expression profile of tumour antigens [40] , possibly preventing also peripheral mechanisms of immune tolerance, such as the broad presentation of TAAs by non-professional antigen presenting cells (APC). This hypothesis is in agreement with the better clinical outcome of patients with tumours displaying a higher density of TLS. However, as this protective effect was necessarily established after resection of TLS-containing tumours, these structures may not be directly involved in survival. It is rather conceivable that this alternative priming of adaptive responses may result in the induction of a more effective cancer-specific lymphocyte memory able to better control dissemination of micrometastases on surgical cancer resection. In accordance with our current results, in an experimental model of melanoma, tumour rejection was promoted by cells expressing NKp46 and depending on the transcription factor RORγt [57] . It should be mentioned, however, that activation of NCR + ILC3 within tumours might not always represent a favourable event: a negative effect in colorectal cancer has recently been proposed for IL-22, which would act on epithelial cells and induce Stat3 phosphorylation and cell proliferation [49] . In this regard, it might be argued that, as mentioned above, lung tumour NCR + ILC3 produce lower levels of IL-22 as compared with tonsillar and, probably, colon-associated NCR + ILC3. On the other hand, the expression of IL-22 receptors such as IL-22R1 and IL-10R2 can be upregulated by TNF-α, suggesting that IL-22 effects may be amplified by this cytokine [58] , abundantly produced by lung tumour NCR + ILC3 on NKp44 engagement. However, on the basis of the association between the amount of tumour NCR + ILC3 and a more favourable prognosis (that is, their correlation with both TLS density and early stages of disease), we favour the idea of a protective role of this ILC subset in anti-tumour immune response against lung cancer cells. Altogether, our data revealed that NCR + ILC3 are an important cellular component of the lymphocytic infiltrate of lung cancers, where they can directly sense tumour and TA cells present in the cancerous microenvironment, mainly via the NKp44-activating receptor. Cell triggering via NKp44 and/or cytokine receptors may result in a relevant innate source of cytokines involved in leukocyte recruitment, endothelial cell activation and lymphoid organ neogenesis. Both NCR + ILC3 and NKp44 receptor could therefore represent interesting novel therapeutic targets for modulating the immune response against NSCLC. In addition, the identification of NCR + ILC3 in tumour specimens should also be further investigated as a new immunoscore factor possibly helpful in determining the prognosis of patients operated on for lung cancer. Patient selection and samples Samples were obtained from 57 untreated patients, without any other concomitant lung disease, who underwent surgical resection of NSCLC. Of these, 18 patients were in tumour stage I, 19 in stage II and 20 in stage III. The samples were provided by the Biological Resource Center of IRCCS AOU San Martino-IST-Istituto Nazionale per la Ricerca sul Cancro and the study was approved by the Institutional Ethics Committee of the same Institution. Tonsils were obtained from patients undergoing tonsillectomy at the Giannina Gaslini Institute. The relevant Institutional Review Boards approved the study and all patients gave their written informed consent according to the Declaration of Helsinki. Cell isolation and sorting Lung tissue specimens (neoplastic tissue and matched normal lung tissue) were obtained immediately after surgical resection of primary tumours. Both normal and tumour tissues were extensively washed in PBS to remove cell debris and red blood cell aggregates, then the weight was assessed. Samples were then mechanically minced by scissors to obtain small fragments that were enzymatically digested with a cocktail containing DNAse (100 μg ml −1 , Roche), collagenase (1 mg ml −1 , Worthington) and hyaluronidase (1 mg ml −1 , Sigma) in RPMI 1640 supplemented with Pen/Strep for 1.5 h at 37 °C. The suspension was then filtered through a cell strainer and, subsequently, washed by centrifugation in PBS to remove residual enzymes. Whenever possible, an aliquot of the cell suspension was used to evaluate the content of polymorphonuclear leukocytes (PMNs), by flow cytometry (FC) ( Supplementary Fig. 3 ). The tissue-cell suspensions from all the samples were then isolated by Ficoll-Hypaque (Sigma) density gradient centrifugation, to obtain tissue-resident mononuclear cells. Human tonsils were mechanically minced by scissors, then filtered through a cell strainer and, subsequently, the tonsil-mononuclear cells were isolated by Ficoll-Hypaque (Sigma). Whenever possible, matched patient’s blood samples were also collected and mononuclear cells were isolated by Ficoll-Hypaque (Sigma). For flow cytometry sorting of NCR + ILC3 and cNK cell subsets, mononuclear cells derived from tumour specimens or tonsils were labelled with LIVE/DEAD Fixable Aqua Dead dye (Invitrogen, L34957, dil: 1:500), APC-H7-conjugated anti-CD45 (BD, 560178, dil: 1:25), fluorescein isothiocyanate (FITC)-conjugated anti-CD3 (Miltenyi, 130-080-401), anti-19 (Miltenyi, 130-091-328), anti-CD14(Miltenyi, 130-080-701), anti-CD34 (Miltenyi, 130-081-001), anti-BDCA2 (Miltenyi, 130-090-510), anti-CRTH2 (Biolegend, 350108) and anti-ILT3 (LS Bio, LS-C261904) all used at the dil: 1:50, and PE-conjugated anti-NKp46 (Miltenyi, 130-092-607, dil: 1:25), APC-conjugated anti-NKp44 (Biolegend, 325110, dil: 1:25), BrillantViolet 421-conjugated anti-CD117 (BD, 562434, dil: 1:50) and PE/Dazzle-conjugated anti-CD127 (Biolegend, 351336, dil: 1:50) antibodies. Cells were sorted as shown in Fig. 2a on a FACSAria (BD) to >95% purity. Isolation of normal epithelial lung cells was performed by staining the mononuclear cell suspension, derived from the disruption of normal lung specimens, with a mixture of unlabelled anti-E-cadherin monoclonal antibody (Santa Cruz., sc-21791, dil: 1:50) coupled with a FITC-conjugated goat-anti-mouse IgG1 secondary monoclonal antibody (Southern Biotech, 1070-02, dil: 1:100), followed by a mixture of LIVE/DEAD Fixable Aqua Dead (dil: 1:500), APC-H7-conjugated anti-CD45 (dil: 1:25), APC-conjugated anti-Fibroblast (Miltenyi, 130-100-132, dil: 1:25) monoclonal antibodies and then by sorting Live/E-Caderin + cells. Expansion of NCR + ILC3 and cNK cell lines Flow cytometry-sorted NCR + ILC3 and cNK cells were stimulated with irradiated allogeneic peripheral blood mononuclear cells and irradiated 721.221 tumour cells in the presence of PHA (1 μg ml −1 , Life Technologies), IL-2 (100 U ml −1 , proleukin; Chiron) and IL-7 (10 ng ml −1 , Miltenyi). Cytokines were replenished every 2–3 days. Cells were cultured in RPMI 1640 medium (Lonza) plus 1% human AB serum. Cell cultures TA fibroblasts were derived from tumour lung specimens. Briefly, cell suspensions derived from tumour specimens were seeded in six-well tissue plates and cultured in RPMI 1640 medium plus 10% FCS. Wells giving rise to cell populations homogeneously displaying fibroblast cell morphology were selected. Fibroblast cell cultures were further phenotypically characterized and assessed for purity by the analysis of anti-fibroblast antibody (Abcam, ab28244, dil: 1:10). Fibroblasts cell lines were cultured in RPMI medium supplemented with FCS 10% and then used within 15 passages. All the human NSCLC cell lines used in the study (A549, NCI-H1975 and SK-MES1) were purchased from Interlab Cell Line Collection of IRCCS AOU San Martino-IST-Istituto Nazionale per la Ricerca sul Cancro and confirmed mycoplasma free. MSCs and endothelial cell assays Human MSCs were derived from the bone marrow, as previously described [59] . Samples were obtained after the ethical committee approval of the institutional review board of the Giannina Gaslini Institute, Genova, Italy, and parental informed consent in accordance with the Declaration of Helsinki. Briefly, bone marrow cell suspensions were plated at a concentration of 1 × 10 6 cells per ml in 25-cm 2 tissue-culture flasks in Mesencult basal medium supplemented with MSC stimulatory supplements (both from StemCell Technologies). After 24 h, non-adherent cells were removed and fresh medium was added. When the cultures nearly reached confluence, cells were detached by treatment with trypsin/EDTA solution (BioWhittaker, Cambrex) and replated at 5 × 10 5 cells per 75-cm 2 tissue-culture flask. The lymphoid-tissue inducing assay was performed as previously reported [19] . Briefly, MSCs were plated in a 48-well plate at a density of 5 × 10 4 cells per well, NCR + ILC3 were then added at a 1:1 ratio and co-cultured for 4 days in the presence of IL-7 (10 ng ml −1 ). Co-cultures were also performed in the presence of TNFRII- and LTβR-Fc-soluble molecules (both from R&D). ICAM-1 (PE-conjugated, Ancell, 206-050, dil: 1:50) and VCAM-1 (APC-conjugated, BD, 551147, dil: 1:50) expression on MSCs was determined by flow cytometry. Similarly, for the endothelial cell activation test, EA.hy926 (human umbilical vein cell line, ATCC CRL-2922) were plated in a 48-well plate at a density of 5 × 10 4 cells per well and NCR + ILC3 were added at a 1:1 ratio and co-cultured for 4 days in the presence of 10 ng ml −1 IL-7. ICAM-1(PE-conjugated, Ancell, 206-050, dil: 1:50) and VCAM-1(APC-conjugated, BD, 551147, dil: 1:50) expression was determined by flow cytometry. Reverse transcription–PCR RNA was extracted from lysed cells using an RNAeasy micro kit (Qiagen, Hilden, Germany). Complementary DNA was genereted using a RealMasterScript Supermix Kit (5PRIME GmbH). Reverse trascription was performed at 25 °C for 5 min, 42 °C for 30 min and 85 °C for 5 min using 1 μg–10 pg of total RNA. Relative quantitation of gene expression was performed in real-time reverse transcription–PCR with Platinum SYBR Green qPCR SuperMix-UDG (Invitrogen) as the housekeeping gene. Amplifications were performed with a Mastercycler ep realplex (Eppendorf) in a 20-μl final volume, using primers at 300 nM for 40 cycles (15 s at 95 °C, 30 s at 52 °C for LTA, 56 °C for LTB). A dissociation curve was carried out at the end of 40 cycles to confirm specificity of amplification. The following primers were used: glyceraldehyde 3-phosphate forward 5′-GAAGGTGAAGGTCGGAGT-3′, glyceraldehyde 3-phosphate reverse 5′-CATGGGTGGAATCATATTGGAA-3′; LTA forward 5′-CCAGCAAGCAGAACTCA-3′, LTA reverse 5′-ATGGGCCAGGTAGAGTG-3′; LTB forward 5′-AGTGCCCCAGGATCAG-3′, LTB reverse 5′-GCCGACGACACAGTAGAG-3′. Relative expression of each transcript was obtained using the ΔΔCT method. Double immunohistochemistry and quantification of TLSs For NKp46/RORγt double staining, paraffin-embedded lung tissue sections were deparaffinized, treated with H 2 O 2 /3% for 5 min to inhibit endogenous peroxidase and then washed in H 2 O. They were then incubated for 30 min with the first primary antibody (mouse anti-NKp46/NCR1 Ab, R&D System, 195314, conc: 5 μg ml −1 ) followed by detection with the Bond Polymer Refine Detection Kit (Leica Biosystems) according to the manufacturer’s protocol and subsequently incubated for 30 min with the second primary antibody (mouse anti-RORγt Ab, Millipore, MABF81, dil: 1:50) followed by detection with the Bond Polymer Refine Red Detection Kit (Leica Biosystems) according to the manufacturer’s protocol. For the quantification of intratumoral TLSs, for each paraffin-embedded lung tumour, two observers (two expert pathologists trained to identify the pathologic features of NSCLC) selected the tumour section containing a representative area of tumour with adjacent lung parenchyma and the highest density of immune cells on the haematoxylin and eosin-safran-stained tissue section. Intratumoral lymphoid structures were counted in the tumoral areas of the entire tissue section (from 18 to 83 fields, original magnification × 100) and expressed as density of TLS (total number of TLS per field). The necrosis and fibrosis were counted as the percentage of the positive areas among the whole tumour mass. Flow cytometry The following antibodies to human proteins were used. From Miltenyi: FITC-conjugated anti-BDCA2 (dil: 1:100), anti-CD3(dil: 1:100), anti-CD14 (dil: 1:100), anti-CD34 (dil: 1:100), PE-conjugated anti-NKp30 (130-092-483, 1:50), anti-NKp44 (130-092-480, dil: 1:50), anti-NKp46 (dil: 1:50), anti-CD117 (130-091-735, dil: 1:50), anti-CD161(130-092-677, 1:100), VioBlue-conjugated anti-KIR3DL1 (130-095-234, dil: 1:33), VioBright FITC anti-CD19 (130-104-578, dil: 1:100) and APC-conjugated anti-CD66abce (130-093-155, dil: 1:50). From BD Biosciences: FITC-conjugated anti-CD80 (555683, dil: 1:100), PE-conjugated anti-CD25 (555432, dil: 1:50), PC7-conjugated anti-CD16 (557744, dil: 1:100), anti-NKp46 (562101, dil: 1:50), AlexaFluor 647-conjugated anti-CCR6 (560466, dil: 1:40), APC-H7-conjugated anti-CD45, Brillant Violet 421-conjugated anti-CD117 and APC-conjugated anti-VCAM-1. From Biolegend: PerCP-Cy5.5-conjugated-CD127 (351322, dil: 1:100), anti-CD117(313214, dil: 1:100), anti-CRTH2 (350116, dil: 1:40), APC-conjugated anti-NKp44 (dil: 1:50), FITC-conjugated anti-CRTH2 (dil: 1:40), PE/Dazzle-conjugated anti-CD127 (dil: 1:100) and BV711-conjugated anti-CD56 (318336, dil: 1:50). From Ancell: FITC-conjugated/PE-conjugated anti-Perforin (358-040 and 358-050, respectively, dil: 1:75 for both). From other manufacturers: FITC-anti-ILT3 (Lifespan Bio,dil: 1:100), PE-/APC-anti-RORgt (eBioscience, 12–6988 and 17–6988, respectively,dil: 1:100 for both), eFluor-660-anti-CD107a (eBioscience, 50–1079, dil: 1:100), ECD-anti-CD3 (Beckman Coulter, IM2705U, dil: 1:50), PC7-anti-CD56 (Beckman Coulter, A51078, dil: 1:25), FITC-anti-CD94 (R&D Systems, FAB1058F, dil: 1:40) and PE- anti-CXCR5 (R&D Systems, FAB190P, dil: 1:20). LIVE/DEAD Fixable Aqua Dead (dil: 1:500) was also used to exclude dead cells. For NCR ligand staining: in-house prepared soluble Fc-NCRs were used according to the following protocol. Briefly, after incubation with the relevant soluble receptor (used at the concentration of 10 μg ml −1 ), cells were washed and PE-conjugated isotype-specific mouse anti-human antibodies (Southern Biotech, 9040-09, dil: 1:200) were added and incubated for 30 min at 4 °C. Intracellular staining with anti-human Perforin was performed using the Fix/Perm kit by BD Biosciences. Intranuclear staining with anti-human PE- or APC-conjugated RORγt was performed using the Fix/Perm buffer set by Biolegend according to manufacturer’s indications. Samples were then acquired using either Gallios (Beckman Coulter) or MACSQuant (Miltenyi Biotech) cytometers and data analysed by FlowJo xV.0.7 (TreeStar Inc.) or Kaluza 2.1 (Beckman Coulter) softwares. Intracellular cytokine staining Intracellular staining for the detection of cytokines was performed on freshly isolated lymphocytes or in-vitro expanded NCR + ILC3s and cNK cell lines stimulated for 6 h with PMA (10 ng ml −1 ) and ionomycin (500 ng ml −1 ) (both from Sigma), and/or IL-23 (50 ng ml −1 ) or IL-23, and IL-7 and IL-1β (all 50 ng ml −1 , all from Miltenyi) in the presence of GolgiStop plus GolgiPlug (both from BD Biosciences). Alternatively, in-vitro expanded NCR + ILC3s cell lines were stimulated with A549, NCI-H1975, SK-MES-1, sorted epithelial cells from normal lung tissues or with TA fibroblasts for 6 h at 37° in the presence of GolgiStop plus GolgiPlug and anti-NKp44 (clone KS38), -NKp46 (clone KL247) and -NKp30 (clone F252) blocking monoclonal antibodies, all produced in our laboratory. Cells were then fixed/permeabilized using Fix/Perm buffer kit (BD Biosciences) according to manufacturer’s indications. The following antibodies were used: APC-conjugated anti-IFNγ (Miltenyi, 130-091-640), dil: 1:100), anti-IL-17a (Miltenyi, 130-094-519, dil: 1:100), PerCP-eFluor710-conjugated anti-IL-22 (eBioscience, 46–7229, dil: 1:50), eFluor450-conjugated anti-TNF (eBioscience, 48–7349, 1:100), PE-conjugated anti-IL-8 (BD, 554720, dil: 1:100) and anti-IL-2 (BD, 554566, dil: 1:200). Samples were then acquired using either Gallios (Beckman Coulter) or MACSQuant (Miltenyi Biotech) cytometers and data analysed by FlowJo xV.0.7 (TreeStar Inc.) or Kaluza 2.1 (Beckman Coulter) softwares. Cytokine detection in culture supernatants Relevant cytokines (IL-22, IL-8, TNFα, IL-2 and IFNγ) were detected in the culture supernatants by using a Human Premixed Multi-analyte kit (R&D). Samples were then acquired using Magpix (Luminex Corporation). Cytotoxic activity assay A549 cells were incubated with 100 μCi of Na 2 51 CrO 4 for 90 min at 37 °C, extensively washed and finally cultured with the different NK cell populations for 4 h at 37 °C. Microculture supernatants were then collected and radioactivity counted on a gammacounter. ‘Specific’ 51Cr release is calculated on the bases of the ratio ((sample release 2 spontaneous release)/(total release 2 spontaneous release)). Assays were performed in triplicate at the indicated effector-target ratios. Tumour-cell proliferation assay A549 cells (see also ‘Cell cultures’ paragraph above) were plated in a 96-well plate at a density of 1.5 × 10 3 cells per well at day 0 (see also ‘Cell cultures’ paragraph above). After 24 h, NCR + ILC3s or cNK cells were added at different (50:1, 10:1, 5:1, 1:1) lymphocyte:tumour cell ratios and co-cultured for additional 4 days in the presence of 10 ng ml −1 IL-7. After the co-culture, cells were extensively washed with PBS to remove lymphocytes, stained for 30 min with 50 μl of crystal violet and then repeatedly washed with water. Next, cells adherent to the plate were then eluted with 100 μl of elution solution (50% ethanol+0.5% CH 3 COOH) and analysed by a spectrophotometer (595 nm). Chemotaxis and adhesion tests For the chemotaxis test, NCR + ILC3s conditioned medium was prepared by stimulating NCR + ILC3s for 24 h, in RPMI medium without serum, with a mixture of antibodies specific for NKp44 (Z231 clone), NKp30 (7A6 clone), NKp46 (BAB281 clone) (all obtained in our laboratory) in a plate coated with F(ab′)2 fragment goat anti-mouse IgG (R&D Systems). The supernatants were collected and added to the lower compartment of Boyden chambers (50 μl/ per well). Collagen type IV (0.1 mg ml −1 in H 2 O 0.1% CH3COOH) or gelatin (0.05 mg ml −1 in H 2 O)-coated filters with 12 μm pores were used as barrier. Human umbilical vein endothelial cells (ATCC CRL-1730) were then plated in the upper compartment, in serum-free medium (50,000 per 200 μl per well). Cells were incubated for 5 h at 37 °C. At the end of the test, cells were fixed in absolute ethanol and stained with toluidine blue. Unmigrated cells from the upper surface of the filter were eliminated cleaning the filters on filter paper. Migrated cells were quantified by densitometric scanning using the NIH Image freeware software. Chemotaxis tests were run in triplicate and repeated four times. Adhesion test was performed in 96-well plates untreated for cell adhesion that were coated with gelatin (0.05 mg ml −1 in H 2 O) and incubated for 30 min at 37 °C. After gelatin discarding, NCR + ILC3s supernatans (50 μl) (prepared as earlier described) were added in quadruplicate to the wells and incubated for additional 30 min. Human umbilical vein endothelial cells (10,000 per 50 μl serum free medium (SFM) per well) were added to NCR + ILC3s conditioned wells and allowed to adhere for 90 min. At the end of the incubation, cells were washed twice with PBS and fixed/stained with crystal violet solution (4% paraformaldehyde, 30% ethanol, 60 mM NaCl, 5 g l −1 crystal violet in H 2 O). Staining was eluted (50% ethanol, 0.1% CH 3 COOH in H 2 O) and quantified by a spectrophotometer (595 nm). Statistical analysis Statistical significance was determined with Student’s t -test, Wilcoxon signed-rank test or linear regression test. Prism GraphPad (GraphPad Software, Inc.) software was used. How to cite this article: Carrega, P. et al. NCR + ILC3 concentrate in human lung cancer and associate with intratumoral lymphoid structures. Nat. Commun. 6:8280 doi: 10.1038/ncomms9280 (2015).